Diversifying evolution of competitiveness In many species, individuals express phenotypic characteristics that enhance their competitiveness, that is, the ability to acquire resources in competition with others. Moreover, the degree of competitiveness varies considerably across individuals and in time. By means of an evolutionary model, we provide an explanation for this finding. We make the assumption that investment into competitiveness enhances the probability to acquire a high-quality resource, but at the same time reduces the ability of exploiting acquired resources with maximal efficiency. The model reveals that under a broad range of conditions competitiveness either converges to a polymorphic state, where individuals differing in competitive ability stably coexist, or is subject to perpetual transitions between periods of high and low competitiveness. The dynamics becomes even more complex if females can evolve preferences for (or against) competitive males. In extreme cases, such preferences can even drive the population to extinction. Competition is arguably the most important factor structuring the living world. Ecological communities are to a large extent shaped by competition among different species, while intraspecific competition for fitness-enhancing resources is the driving force behind natural selection [1] . Here we focus on competition among the individuals of a species, addressing the question of how much individuals should invest into increasing their competitiveness, that is, the ability to be successful in competition with others. There are many ways how organisms can enhance their competitive ability. Trees produce high stems, thereby outshading competing trees and offering their own leaves a place in the sun [2] , [3] . In competitive environments, guppies (and many other animals) invest in better sensory capabilities to locate food more efficiently than their conspecifics [4] . Male bluegill sunfish grow large to be able to acquire and defend a breeding territory [5] . In other species, individuals grow horns, antlers and other armament for the same purpose [6] . Male sticklebacks develop a red belly to deter other males and to attract females [7] . Virtually all features enhancing competitive ability come at a cost. For example, growing large or developing armament takes time and energy that could otherwise be spent on other activities increasing Darwinian fitness. Moreover, there is often a trade-off between being able to acquire many or high-quality resources and the ability to make best use of these resources. For example, trees allocating much energy into the production of a large stem achieve a good position in the light gradient, but they can allocate less energy into the production of leaves and hence are less able to exploit this good position [2] . Sticklebacks with a red belly attract many females and therefore have many eggs in their nest, but they also attract predators [8] , reducing the survival probability of these eggs. Red-legged male Zebra finches attain many extra-pair copulations but invest less into paternal care, thus achieving a lower reproductive success with their social mate [9] . In view of these costs and trade-offs one might expect a single optimal level of investment in competitiveness, at which the benefits of a higher competitive ability are balanced by the associated costs. In contrast to this expectation, there is compelling evidence from many organisms that members of the same population differ considerably in the degree they allocate energy and resources into enhancing their competitive ability. Trees, for example, differ in their relative investment into stem versus leaves; some trees outgrow their competitors by producing a large stem, while others remain in shadow but make better use of light of lower intensity [2] , [3] . Only a fraction of male bluegill sunfish grows large to become good competitors for territories; the remainder stops growing early on and attains an alternative mating strategy [5] . Similarly, a ‘pace-of-life syndrome’ is found in many species: some individuals invest heavily into obtaining favourable reproductive positions (for example, a high position in a dominance hierarchy), while others consistently avoid risks and seem to be content with a lower position [10] , [11] . In addition to such coexistence of individuals differing in competitiveness, the overall degree of competitiveness may also vary considerably in space and time. For example, temporal cycles in aggressiveness (associated with competitive ability) have been reported in many rodent species [12] , [13] , while spatial waves of aggressiveness have been observed in other species, for example, Western bluebirds [14] . In side-blotched lizards, the relative abundance of three male morphs differing in competitiveness exhibits both variation in space and oscillations in time, with the high-competitive orange morph predominating in some years and the less-competitive yellow and blue morphs predominating in others [15] . To achieve a better understanding of these patterns, we investigate a model that captures essential features of the evolution of competitiveness. We assume that individuals compete for a spectrum of resources varying in quality. Each individual can allocate a fraction c of its energy into enhancing its competitiveness. Individuals with higher competitiveness attain on average higher-quality resources than individuals with lower competitiveness. To incorporate the costs of competitiveness and to address the fact that high-competitive individuals can often not make maximal use of their resources, we assume that reproductive output of an individual is proportional to (1− c ) R , where c is the competitiveness of the individual and R is the quality of the resource obtained by this individual. This formulation encapsulates the basic trade-off between the ability to acquire resources (a high value of c is associated with a high value of R ) and the ability to exploit the acquired resources (an individual with a lower value of c extracts more ‘value’ out of a given resource R than an individual with a higher value of c ). We first consider a baseline scenario where the individuals of a population compete for resources that are either of high or of low quality. Individuals with higher competitiveness have a higher probability to acquire a high-quality resource. Evolutionary simulations reveal that the population will either evolve to a polymorphic state (where individuals of low competitiveness coexist with individuals of high competitiveness) or that the population exhibits regular cycles between low and high competitiveness. The evolutionary outcome depends on two factors: the difference in resource quality and the extent to which the acquisition of high-quality resources depends on stochastic factors (in addition to competitiveness). These conclusions are confirmed and quantified in a mathematical analysis that is based on an adaptive dynamics approach. The analysis reveals that, interestingly, polymorphism does not arise by ‘evolutionary branching’ [16] , but in a more intricate manner. By means of additional simulations, we show that the conclusions of our highly simplified baseline model extend to other scenarios, such as a continuous distribution of resource qualities. We then expand the model by allowing the evolution of female preferences for male competitiveness or, more indirectly, for the quality of resources acquired by potential mates. With this addition, the evolutionary dynamics becomes even more complex. Preferences can also be polymorphic and subject to perpetual change. Females often prefer highly competitive males although less-competitive males provide more paternal care. Such preferences can even drive the population to extinction. Evolutionary dynamics of competitiveness We first report on individual-based evolutionary simulations for our baseline scenario. The individuals of a population compete for a resource that occurs in two qualities, R low and R high . Each individual i is characterized by an inherited competitiveness value c i that is transmitted from parents to offspring subject to rare mutations. Realized competitiveness is given by c i + ε , where ε is a random variable taking account of all kinds of stochastic factors affecting success in resource competition. Individuals with above-average realized competitiveness receive a resource of high quality ( R i = R high ), while the others receive a resource of low quality ( R i = R low ). The number of offspring produced by individual i is proportional to (1− c i ) R i . After reproduction, the parental generation dies and is replaced by their offspring. The simulations in Fig. 1 are representative for the evolutionary outcome of this model. When the variation in resource qualities is small (left panel), the system converges to a stable polymorphism, where part of the population attains an intermediate level of competitiveness while the remainder is not competitive at all. When the variation in resource quality is large (right panel), we observe a strong temporal dynamics: when competitiveness is low it gradually increases to very high levels; but once such a high level is reached, competitiveness collapses to a low level and the cycle starts again. The rapid turnover of competitiveness strategies can be understood as follows. As long as the population is monomorphic for one level of competitiveness, any mutation inducing a small increase in this level has a large fitness advantage (since mutants receive the high-quality resource), leading to the spread of this mutation. This results in an arm’s race to ever higher levels of competitiveness. The race is, however, stopped when competitiveness reaches very high levels and low-competitiveness mutants arise. In fact, a high degree of competitiveness c high is associated with a low value of (1− c high ), implying that the resulting fitness (1− c high ) R is small even if a high-quality resource can be acquired ( R = R high ). A mutant with competitiveness c low will only get access to a low-quality resource, but still its fitness (1− c low ) R low can be considerably higher. As a consequence, the mutants will spread and oust the resident population. 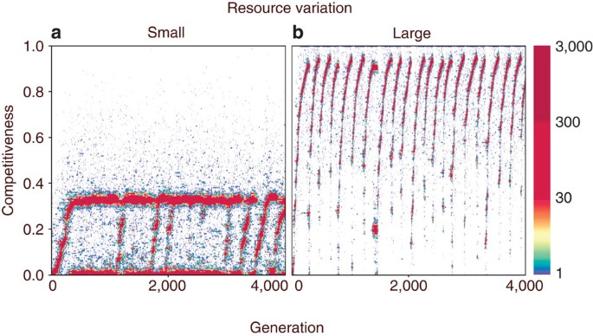Figure 1: Evolutionary dynamics of competitiveness. Individuals of high competitiveness have a higher chance of obtaining a high-quality resource, but they cannot exploit the resource obtained with maximal efficiency. When variation in resource quality is small ((a);Rlow=0.8,Rhigh=1.2) the population is dimorphic most of the time, consisting of individuals with low competitiveness and individuals with intermediate competitiveness. Turnovers between low and intermediate competitiveness occur once in a while. When variation in resource quality is large ((b);Rlow=0.2,Rhigh=1.8) the population exhibits regular cycles between low and high competitiveness. Figure 1: Evolutionary dynamics of competitiveness. Individuals of high competitiveness have a higher chance of obtaining a high-quality resource, but they cannot exploit the resource obtained with maximal efficiency. When variation in resource quality is small (( a ); R low =0.8, R high =1.2) the population is dimorphic most of the time, consisting of individuals with low competitiveness and individuals with intermediate competitiveness. Turnovers between low and intermediate competitiveness occur once in a while. When variation in resource quality is large (( b ); R low =0.2, R high =1.8) the population exhibits regular cycles between low and high competitiveness. Full size image Occasionally, similar cycles also occur in case of polymorphic populations that are seemingly in equilibrium ( Fig. 1 , left panel). Conversely, the population can remain polymorphic while competitiveness cycles between very low and very high levels. Examples for both outcomes will be discussed in Supplementary Figs 1 and 2 . These figures also illustrate that polymorphisms and cycles in competitiveness are also obtained in diploid populations and in case of a continuous spectrum of resources. Analysis based on fitness considerations To get a better idea under which circumstances polymorphism and cycles are to be expected, we applied an adaptive dynamics analysis to our baseline model (see Methods). To simplify the analysis, we assumed that the stochastic term ε is uniformly distributed over the interval [− s , + s ]. As shown in the methods, the evolutionary outcome strongly depends on three model parameters: the degree s to which the acquisition of high-quality resources is determined by chance, the average resource quality R m =½( R high + R low ) and the variation in resource quality Δ= R m − R low . If s >Δ/ R m , competitiveness does not get off the ground and the population converges to c *=0. Apparently, it does not pay to invest in competitiveness if the outcome of competition is strongly determined by stochastic effects or if the difference in resource quality is very small. If s <Δ/ R m , there is an intermediate level of competitiveness 0< c *<1 that is evolutionarily stable and convergence stable and, hence, an evolutionary attractor [16] , [17] . Yet, if much is at stake (Δ is large) and competitive success is more strongly dependent on competitiveness than on stochastic factors ( s is small), a monomorphic population with competitiveness c * is not the end point of evolution. In fact, such a population can be destabilized by the advent of mutants with low competitiveness if . If in addition s >( R m −Δ)/( R m +Δ) 2 , the population typically ends up in a dimorphic state where a high-competitive genotype coexists with the non-competitive genotype c =0. Otherwise (if s <Δ( R m −Δ)/( R m +Δ) 2 ), this dimorphism gets destabilized as well, resulting in perpetual cycles in competitiveness (see Supplementary Fig. 3B ). The parameter domains corresponding to the four qualitatively different types of model behaviour are depicted in Supplementary Fig. 4 . Simulations incorporating the assumptions of the mathematical analysis (that is, with a uniformly distributed stochastic term ε ) fully confirm the above conclusions (see Supplementary Fig. 5 ). Evolution of female preferences for competitive males In many organisms, males are more competitive than females. Males compete for access to resources, while females are choosy with whom to mate [18] . In situations where females directly benefit from the resources available to their mate (for example, if the mates allocate these resources to paternal care), one would expect that females make their choice of a mate in one way or the other dependent on the quality of these resources. To model the evolution of female preferences, we consider a population with two sexes. Only males compete for resources, and competitiveness c is only expressed in males. Female preferences are based on the resource quality obtained by potential mates and characterized by a heritable parameter p . Females with a positive value of p prefer to mate with males having acquired above-average resources, while females with a negative value prefer males with below-average resources. The absolute value of p determines the strength of the preference. In the Supplementary Material we also consider the scenario where female preferences are not based on resource quality but more directly on male competitiveness. 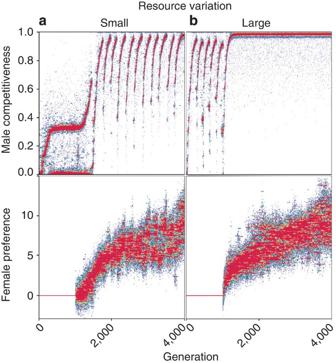Figure 2: Joint evolution of male competitiveness and female preferences based on male resources. After 1,000 generations of evolution in the absence of female choice (p=0, resulting in a dynamics as inFig. 1), female preferences are allowed to evolve. In the standard version of the model, female always evolve a strong preference for males with high-quality resources (p>0), thereby favouring males of higher competitiveness. In case of small variation in resource quality ((a);Rlow=0.8,Rhigh=1.2) polymorphism gives way to large-amplitude cycles in male competitiveness. In case of large variation ((b);Rlow=0.2,Rhigh=1.8) the cycles disappear and male competitiveness evolves to a maximal level. Figure 2 shows the effect of female choice in the case of small (left panels) and large (right panels) variation in resource quality. For the first 1,000 generations, female preference p was kept fixed at p =0, corresponding to random mating. Thereafter, p was free to evolve. In the standard version of our model, female preferences always evolve to high positive values. In other words, females evolve a strong preference for above-average resources, thereby enhancing the selection pressure on males to acquire such resources. As a consequence, even in case of small variation in resource quality (left panels) males are forced into competitiveness cycles, while in case of large variation male competitiveness is driven to almost maximal levels. As shown in Supplementary Figs 6–8 , these conclusions not only apply to the standard version of our model, but also to other distributions of resource qualities and under other assumptions on the action of sexual selection and on the inheritance of competitiveness and preferences. From the perspective of individual selection, the evolution of preferences for high-quality resources is understandable, since, all other things being equal, females profit from such resources. From a population perspective, however, this outcome is highly disadvantageous. In fact, competitive individuals ‘waste’ part of the resources they acquire, and only a non-competitive population makes maximal use of the resources available. 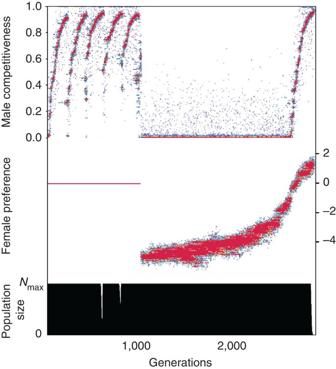Figure 3: Evolutionary suicide caused by the evolution of female preferences for high-quality resources. In the first 1,000 generations, male competitiveness evolves in the absence of female preferences (p=0) in a scenario with large variation in resource quality (Rlow=0.2,Rhigh=1.8). In contrast to the earlier simulations female productivity is limited (60 eggs per female), resulting to a pronounced decline in population size when male competitiveness gets too high (generations 580 and 780). From generation 1,000 onwards, female preferences can evolve, starting from a negative value (p=−5). As long as preferences stay negative, male competitiveness remains low, resulting in an ecologically favourable state where no resources are wasted for competitiveness. However, female preferences evolve to positive values; this induces the evolution of male competitiveness to very high levels, eventually causing population extinction. Figure 3 illustrates these negative implications of a race to ever higher levels of competitiveness. Up to now, we kept population size constant, implying that on average each pair of individuals produces two surviving offspring, irrespective of whether these individuals make prudent use of their resources or not. When the ecological conditions are harsh, this assumption is not realistic. We therefore modified the model by limiting the number of offspring produced per female and assuming that the survival probability per offspring is proportional to the amount of paternal care provided by the female’s mate (which in turn is proportional to (1− c ) R ). Now the population can decline if competitiveness is too high and, accordingly, offspring survival is too low. Figure 3 shows the effects of the joint evolution of male competitiveness (top panel) and female preferences (middle panel) on population size. In the absence of female preferences (first 1,000 generations), the characteristic cycles in male competitiveness can lead to a considerable decrease in population size in those periods where competitiveness is particularly high. When females are in favour of males with a low-quality resource ( p <0; generations 1,000 till 2,800), male competitiveness stays close to zero, no resources are wasted and the population remains at its carrying capacity. Eventually, however, females evolve preferences for high-quality resources, thus fuelling the males’ race towards ever higher levels of competitiveness. In the simulation shown, this results in ‘evolutionary suicide’ [19] : population extinction caused by selection where obtaining an individual fitness advantage is associated with a loss of productivity at the population level. Figure 2: Joint evolution of male competitiveness and female preferences based on male resources. After 1,000 generations of evolution in the absence of female choice ( p =0, resulting in a dynamics as in Fig. 1 ), female preferences are allowed to evolve. In the standard version of the model, female always evolve a strong preference for males with high-quality resources ( p >0), thereby favouring males of higher competitiveness. In case of small variation in resource quality (( a ); R low =0.8, R high =1.2) polymorphism gives way to large-amplitude cycles in male competitiveness. In case of large variation (( b ); R low =0.2, R high =1.8) the cycles disappear and male competitiveness evolves to a maximal level. Full size image Figure 3: Evolutionary suicide caused by the evolution of female preferences for high-quality resources. In the first 1,000 generations, male competitiveness evolves in the absence of female preferences ( p =0) in a scenario with large variation in resource quality ( R low =0.2, R high =1.8). In contrast to the earlier simulations female productivity is limited (60 eggs per female), resulting to a pronounced decline in population size when male competitiveness gets too high (generations 580 and 780). From generation 1,000 onwards, female preferences can evolve, starting from a negative value ( p =−5). As long as preferences stay negative, male competitiveness remains low, resulting in an ecologically favourable state where no resources are wasted for competitiveness. However, female preferences evolve to positive values; this induces the evolution of male competitiveness to very high levels, eventually causing population extinction. Full size image Fortunately, the implications of the evolution of competitiveness on population survival are not always as disastrous as Fig. 3 suggests. When the variation in resource quality is small or the productivity per female is high, the effects on population size will be much smaller. 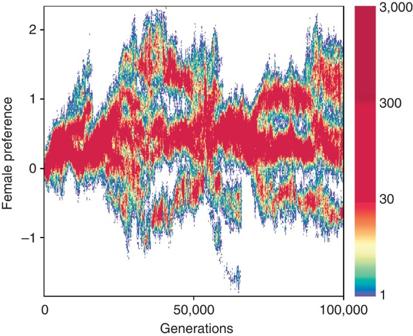Figure 4: Long-term evolution of female preferences. While female preferences always increase in the haploid version of the model, they tend to diversify in the diploid version (shown here). Over long periods of time, three types of females coexist: females with a strong preference (p>1) for high-quality resources, females with a weaker preference (0<p<1) for such resources and females with a preference for low-quality resources (p<0). Figure 4 illustrates that the effects of the evolution of competitiveness on population persistence are also smaller in the diploid version of our model. Also in this case, female preferences evolve on average to positive values, inducing males to evolve higher levels of competitiveness (see Supplementary Figs 9 and 10 ). Now, however, the female population is polymorphic as well, with opposite preferences coexisting in the same population. The fact that a fraction of females has a preference for low-quality resources limits the race towards higher levels of competitiveness, thus leading to a more prudent use of resources at the population level. Figure 4: Long-term evolution of female preferences. While female preferences always increase in the haploid version of the model, they tend to diversify in the diploid version (shown here). Over long periods of time, three types of females coexist: females with a strong preference ( p >1) for high-quality resources, females with a weaker preference (0< p <1) for such resources and females with a preference for low-quality resources ( p <0). Full size image By means of a simple model, we have demonstrated that the evolutionary dynamics of competitiveness can be surprisingly complex. The model predicts both the coexistence of different competitiveness strategies and the high temporal dynamics of competitiveness observed in many organisms. In general, female choice drives the evolution of male competitiveness to higher levels, although highly competitive males waste part of their resources and, therefore, provide less parental care or other direct fitness benefits than could have provided with a lower investment in competitiveness. The model shows that the race towards ever higher levels of competitiveness, which is partly fuelled by female preferences, can make a population very vulnerable and even lead to population extinction. Our model also exemplifies that even in competitive societies males of low competitiveness and females with a preference for such males can stably persist: such individuals tend to acquire lower-quality resources, but they compensate for that by making more efficient use of these resources. Last, but not least, our model also suggests an explanation for spatial variation in competitiveness: if the competitiveness cycles at different locations run out of phase, the degree of competitiveness may differ considerably between these locations. Both in ecological and evolutionary theory the question of competitive coexistence has received a lot of attention. In ecology, the resource competition theory predicts that competing species can stably coexist if they differ in resource consumption patterns and their resource requirements [20] , [21] , [22] . The dynamics of resource competition can be highly complex and lead to perpetual oscillations or chaos [22] , [23] , [24] , [25] , [26] and to spatial patterning of communities [27] . Our model differs from ecological competition models in at least two important ways. First, we consider intraspecific competition rather than competition among species. As a consequence, the competitors in our model (different genotypes) are quite similar to each other, while most ecological models presuppose that there are distinct differences between competing species [28] . Second, the ecological resource competition theory tends to focus on the ‘technologies’ to make the most efficient use of the available resources; if a better competitor arises, more or different resources become available due to improved technologies to locate, extract and consume resources, and to turn resources into biomass production. In contrast, we consider the situation where a higher competitive ability does not make new resources available, but mainly leads to a more favourable outcome in the distribution of a fixed spectrum of resources over organisms. For example, in the context of light limitation we would think of the competition for achieving the best spot in the light gradient [29] , rather than competition for making the most efficient use of light or for making use of those parts of the light spectrum that are left unexploited by competitors [30] . Our model is in the tradition of (evolutionary) models of interference competition, where individuals compete for access to a limited number of high-quality breeding or feeding sites [31] , [32] , [33] . Many models have been developed on the evolutionarily stable strategy in such a competitive context [34] , [35] , [36] , [37] , [38] , [39] , [40] . The majority of these models is based on a limited number of discrete strategies, while our model considers a continuum of strategies. Our model is more related to evolutionary games such as ‘war of attrition’ [34] , [41] , [42] , where the strategy space is also continuous and where a small change in competitive effort can have a major effect on competitive success. The new feature of our model is the assumption that the costs of competitive effort are related to a lowered ability to make best use of the acquired resources. Typically, an adaptive dynamics approach [16] , [17] is the method of choice when analysing adaptive evolution in case of a continuum of competitive strategies. Adaptive dynamics theory has shown how polymorphism can emerge in such a scenario by ‘evolutionary branching’ [16] , [43] . Different competitive strategies can, for example, coexist if the resource utilization ability of each strategy is narrower than the resource distribution [44] , [45] . In our model, competitive coexistence and competitive cycling are not caused by evolutionary branching. In fact, an adaptive dynamics analysis not accompanied by a simulation study might have concluded that the population would always converge to the unique evolutionary attractor c *. Our study exemplifies that, as in other models [39] , [46] , [47] , evolutionary branching is not the only evolutionary route to polymorphism. Evolutionary branching is based on the assumption that mutations have an infinitesimal phenotypic effect. In our simulations, mutational effect sizes are drawn from a normal distribution with small s.d. As a consequence, mutations typically have a small effect, but once in a while mutations of larger effect do occur. As we have shown, such mutations can destabilize the evolutionary attractor c * and induce polymorphism or cycling. To speed up this process, we occasionally allowed for mutations of somewhat larger effect size. We do not consider this assumption unrealistic, since the limited available evidence suggests that in natural populations mutational distributions have fat tails, implying that mutations with larger effect are not uncommon [48] , [49] . Moreover, even from a gradualist perspective it seems plausible that ‘loss-of-function’ mutations will regularly occur, since there are many ways how random mutations can hamper the development of a complexly designed phenotypic trait. If we may view the genotype c =0 (zero competitiveness) as such a loss-of-function mutation, just that mutation would be most likely that most efficiently triggers the evolution of polymorphism or cycling. We conclude that in models with a continuum of strategies, evolutionary branching should be viewed as a worst-case scenario for the emergence of polymorphism and that other routes to the coexistence of competitive strategies deserve serious consideration. General assumptions The individuals in our model compete for resources that are essential for their reproduction. These resources differ in quality. In our standard scenario, we consider the situation where there are two resource qualities R low = R m −Δ and R high = R m +Δ occurring with equal probability. Hence, R m is the mean resource quality, while Δ quantifies the variation in resource quality. Our results do not change if all resource qualities are rescaled by dividing them by a common factor (for example, by R m ). In all simulations, we therefore assume, without loss of generality, that R m =1. The analysis of the situation that the abundances of R low and R high differ is beyond the scope of this paper. Analytical results and extensive simulations (to be published elsewhere) suggest that all outcomes reported here also apply to scenarios where the abundances of resource qualities differ. The robustness of our conclusions is further supported by Supplementary Figs 1 and 6–8 , which consider the alternative scenario that resource qualities are uniformly distributed over the interval [ R m −Δ, R m +Δ]. Each individual has a genetically determined degree of competitiveness c (0≤ c ≤1). Individuals with high competitiveness tend to acquire resources of high quality, but the allotment of resources to individuals is also affected by stochastic effects. To model this, we assume that ‘realized’ competitiveness is given by c r = c + ε , where ε is a stochastic error term. In our standard scenario, 50% individuals with highest realized competitiveness acquire resources of quality R high while the other 50% receive resources of quality R low . In the mathematical analysis, we make the simplifying assumption that ε is drawn from a uniform distribution on the interval [− s , + s ]. This implies that the s.d. of the error term is . In the simulations, we make the more realistic assumption that ε is normally distributed with mean zero and s.d. σ ε . Additional analyses and additional simulations revealed that the distribution of the error term does not affect the main conclusions of this study (see Supplementary Figures ). We assume that there is a trade-off between the ability to acquire high-quality resources in competition with conspecifics (that is, competitiveness) and the ability to exploit the acquired resources with maximal efficiency. If R denotes the resource acquired by an individual with competitiveness c , then a fraction (1− c ) R of this resource can actually be utilized for the production of offspring. Adaptive dynamics analysis For the invasion analysis, we need to determine the fitness w ( c , ĉ ) of a rare mutant with competitiveness c in a resident population with competitiveness ĉ . This is given by , where is the expected resource quality obtained by a c -individual in a ĉ -population. The probability that a c -mutant obtains a high-quality resource equals the probability that it has a higher realized competitiveness than the population average ĉ . Since the realized competitiveness of the mutants is uniformly distributed over the interval [ c − s , c + s ], this probability is 0 if c < ĉ − s , it is 1 if c > ĉ + s and it is if . This implies that is equal to R low if c < ĉ − s , equal to R high if c > ĉ + s and if . Multiplying with (1− c ) yields invasion fitness. In particular, if . The pairwise invasibility plots [16] , [17] in Supplementary Fig. 3 are based on this fitness function. We analyse the fitness function by means of a standard adaptive dynamics approach [17] . The selection gradient is given by . Equalizing this with zero yields the unique interior evolutionarily singular strategy c *=1− R m s /Δ (which satisfies 0< c *<1 if s <Δ/ R m ). A straightforward calculation shows that c * is evolutionarily stable and convergence stable and, hence, an evolutionary attractor. In particular, evolutionary branching [16] does not occur, and polymorphism does not arise via the repeated invasion of mutations with infinitesimally small effect. However, as shown earlier in other models [39] , [46] , [47] , evolutionary branching is not necessarily a prerequisite for the evolutionary emergence of polymorphism. In the next section, we will sketch how polymorphism arises in our model. If s is sufficiently small or Δ is sufficiently large, the monomorphism c * is only locally stable (see Supplementary Fig. 3B ). In fact, a mutant with competitiveness zero can invade a c *-population if or, equivalently, if . Although the advent of the genotype c =0 can lead to the collapse of the monomorphism c *, a population consisting of c =0 individuals is not stable either. As illustrated by the pairwise invasibility plots in Supplementary Fig. 3 (and the simulations in Supplementary Fig. 5 ), genotypes with higher and higher competitiveness will get established by a sequence of gene-substitution events. This process will, however, stop before the evolutionarily stable and convergence-stable genotype c *=1− R m s /Δ is reached. In fact, a stable dimorphism of the zero-competitive genotype c =0 with a genotype of higher competitiveness c h will get established if c h satisfies the condition Δ/ R m < c h <2Δ/ R high . This can be seen as follows: a straightforward calculation shows that both genotypes have the same fitness if the frequency p h of c h in the dimorphic population is equal to either or . These equilibrium frequencies satisfy . Genotype c h has a higher fitness than c =0 if, and only if, . Hence, c =0 will spread when rare in the c h -population until a stable dimorphism of both genotypes is reached where the frequency of c h is equal to . Notice that this dimorphism is stable without satisfying the condition mutual invadability: while c =0 will spread when rare in a c h -population, the opposite is not the case (since c h has lower fitness than c =0 if and, in particular, in a monomorphic c =0 population). Accordingly, a dimorphism will only appear after the previous establishment of a monomorphism with c h >Δ/ R m via a sequence of gene-substitution events. The establishment of a dimorphism of c h and c =0 is not necessarily the end point of evolution. On a longer-term perspective, the dimorphism can be destabilized by the advent of a mutation c k ≠ c h . The fitness of such mutants is (as long as the mutant is rare), where is the average quality of resources acquired by c h -individuals. A mutant will invade if w poly ( c k , c h )> w poly ( c h , c h ). Invasibility can again be judged by investigating the selection gradient . The result is that the dimorphism of c =0 with is evolutionarily stable and convergence stable, that is, an evolutionary attractor. In other words, if , the system has (at least) two locally stable attractors: a monomorphic population with competitiveness c *=1− R m s /Δ and a dimorphic population where individuals with competitiveness c =0 coexist with individuals with competitiveness . One restriction needs to be made: if (which happens if ), the frequency of high-competitive individuals in the dimorphic equilibrium is smaller than ½. In that case, a fraction of the non-competitive individuals will obtain the high-quality resource. As a consequence, the genotype c =0 will be invaded by mutants with a slightly higher competitiveness, which obtain the high-quality resource at minimal cost. A situation such as this will result in evolutionary cycles: a high-competitive monomorphic equilibrium can be invaded by low-competitive mutants, but these mutants can in turn be invaded by genotypes of higher competitive ability (see Supplementary Fig. 3B ). Individual-based simulations The standard versions of our model are based on a fixed population size of N individuals (asexual reproduction) or N males and N females (sexual reproduction). In all figures shown, N =3,000. Generations are discrete and non-overlapping. At the start of each generation, resources are assigned to competing individuals as follows. First all individual i are assigned a realized competitiveness value c i + ε by adding a randomly drawn number ε to i ’s genetic competitiveness value c i . In our baseline model, all individuals with above-average realized competitiveness receive a resource of quality R high while the other individuals receive a resource of quality R low . In the model variants with a continuous distribution of resource qualities, N resources are drawn at random from this distribution. The N individuals are ranked according to realized competitiveness, and the N resources are ranked according to resource quality. Each individual i receives that resource R i which matches in rank individual i ’s competitiveness rank. In case of asexual reproduction, each individual produces on average n (1− c i ) R i offspring, where n is chosen large enough to ensure that the total number of offspring produced is larger than N . Subsequently the parental population is replaced by N new individuals that are drawn at random (without replacement) from the offspring produced. In case of sexual reproduction, each female chooses one mate as a parent for her offspring; each male can be chosen by several females. Together a pair produces on average n (1− c i ) R i surviving offspring, where n is chosen large enough to ensure that the total number of surviving offspring is larger than 2 N . Subsequently the parental population is replaced by N new males and N new females that are drawn at random from the surviving offspring. (Our results are not affected by deviations from a 1:1 sex ratio.) To ensure a constant population size, clutch size n had to be adapted to the average value of (1− c ) R in the population. In contrast, n was kept fixed in the ‘evolutionary suicide scenario’ of Fig. 3 , leading to a decline in population size when the average value of n (1− c ) R turned out to be smaller than two. In the version of the model with two sexes females can exert mate choice based on either the quality of the resource acquired by potential mates or by the competitiveness of potential mates. In line with standard models of sexual selection [50] , the direction and strength of female preference is characterized by a heritable trait p . When preference is based on resource quality, the probability of choosing a particular male as mate is given by the logistic expression , where R is the quality of the resource acquired by the male, is the average resource quality, and α is a scaling factor that has no effect on the direction of evolution. δ is a stochastic error term (drawn from a normal distribution with mean zero and s.d. σ δ ) that takes account of the fact that females may not be able to judge a male’s resource quality with perfect accuracy. The case p =0 corresponds to random mating, since all males have the same probability of being chosen. If p >0 males with (perceived) above-average resources have a higher probability of being chosen, while males with below-average resources are preferred as mates if p <0. When female preferences are based on competitiveness, the probability that a male with competitiveness c is chosen as mate is likewise given by , where is the average competitiveness in the population. In both scenarios, each female selects one male as a mate and produces one clutch of n offspring. The survival probability of each offspring is proportional to (1− c ) R , where c and R are the competitiveness and the quality of the acquired resource of the female’s mate, respectively. The individuals of our model harbour two gene loci with infinitely many alleles per locus. The c -locus determines competitiveness and is only expressed in males. The p -locus determines female preference and is only expressed in females. In the haploid version of our model, each individual harbours one c -allele and one p -allele. The values of these alleles correspond directly to the individual’s competitiveness or preference. The haploid offspring genotype is determined by independently drawing a c -allele and a p -allele from the alleles of its parents, where paternal and maternal alleles are drawn with the same probability. In the diploid version of the model, each individual harbours two alleles at each locus. We assume that the alleles per locus have additive effects on the phenotype. In other words, the phenotypic value of competitiveness and preference are given by the arithmetic mean of the two allelic values at the corresponding locus. The offspring genotype is determined in a standard Mendelian way: at each locus, one allele is randomly chosen among the alleles of the mother, while the other allele is chosen among the alleles of the father. The two loci are unlinked (corresponding to being located on different chromosomes), because the allotment of alleles at one locus is independent of the allotment at the other locus. All these assumptions reflect standard assumptions of sexual selection theory; the implications of these assumptions on the outcome of sexual selection is discussed in ref. 50 . After the offspring have received their alleles from their parents, a mutation can occur with a small probability μ c (resp. μ p ) per locus. In such a case, a randomly chosen number ε is added to the original allelic value, where the mutational step size ε is drawn from a normal distribution with mean zero. Most mutational steps are drawn from a distribution with a small s.d. σ c (resp. σ p ), but occasionally (with probability π c resp. π p ) mutational steps are drawn from a distribution with a larger s.d. σ c + (resp. σ p + ) (see the Discussion section for a justification). We ran at least 50 simulations for each variant of the model and for each parameter setting. Since the simulation outcomes were highly repeatable, we only show a single representative simulation run per setting. The results reported here are based on R m =1 and Δ=0.2 (small resource variation) and Δ=0.8 (large resource variation), respectively. The scaling factor α was set to 2.5; any other value would have led to identical results, up to a proportionate change in the scale of p . The s.d. of the error terms ε and δ were set to σ ε = σ δ =0.01. Mutation rates were relatively large ( μ c = μ p =0.01), but this was compensated by the fact that mutational step sizes were typically rather small ( σ c =0.01, σ p =0.5). Somewhat larger mutational steps occurred with π c = π p =0.1 and s.d. σ c + =0.2, σ p + =1.0. To prevent too rapid evolution of female preferences in Figs 3 and 4 , the mutational step size at the preference locus were reduced to σ p =0.1 and σ p + =0.2 in Fig. 3 and to σ p =0.05 and σ p + =0.1 in Fig. 4 . All results reported are robust with respect to a change in mutation rate and/or mutational step size. Roughly speaking, the time scale of change is proportional to the mutation rate and to the mutational variance (the square of the s.d. of distribution of step sizes). Hence, reducing the mutation rate by a factor 2 retards the simulation by the same factor, while reducing the s.d. of the step size distribution by a factor 2 reduces the speed of evolution by a factor 4. How to cite this article: Baldauf, S. A. et al . Diversifying evolution of competitiveness. Nat. Commun. 5:5233 doi: 10.1038/ncomms6233 (2014).